A bimetallic nanoantenna for directional colour routing Recent progress in nanophotonics includes demonstrations of meta-materials displaying negative refraction at optical frequencies, directional single photon sources, plasmonic analogies of electromagnetically induced transparency and spectacular Fano resonances. The physics behind these intriguing effects is to a large extent governed by the same single parameter—optical phase. Here we describe a nanophotonic structure built from pairs of closely spaced gold and silver disks that show phase accumulation through material-dependent plasmon resonances. The bimetallic dimers show exotic optical properties, in particular scattering of red and blue light in opposite directions, in spite of being as compact as ∼ λ 3 /100. These spectral and spatial photon-sorting nanodevices can be fabricated on a wafer scale and offer a versatile platform for manipulating optical response through polarization, choice of materials and geometrical parameters, thereby opening possibilities for a wide range of practical applications. Noble metal nanoparticles support surface plasmon resonances, collective oscillations of surface electrons that provide means to manipulate light at the nanoscale. Plasmonic nanomaterials are promising components in emerging technologies for improved photovoltaic [1] and biosensing [2] , [3] devices and they have long been known for their ability to generate strong optical near-fields [4] , enabling a family of surface-enhanced molecular spectroscopies that include surface-enhanced Raman scattering [5] and enhanced fluorescence [6] . Nanoplasmonic structures have also been used to control the polarization and propagation direction of light emitted by individual quantum sources [7] , [8] , [9] , [10] , to generate strong optical non-linearities [11] and as a basis for negative-index meta-materials for optical frequencies [12] , [13] , [14] , [15] , [16] . The latter application, as well as directional optical antennas [9] , [17] , [18] and Fano resonant structures [19] , [20] , [21] , typically requires coherent oscillations of several dipolar plasmonic oscillators with specific phase retardations. For example, artificial magnetic dipoles used to induce negative refraction can be based on antisymmetric plasmon modes in dimers, that is, two coupled dipoles oscillating with an internal phase shift of 180° [13] , [22] , [23] , whereas directional emission from nanostructures typically use spatial phase retardation between nearby dipolar antenna elements. However, in all the cases, the phase optimization process involves both spectral tuning of the plasmon resonance and spatial tuning of the device geometry, which requires very precise nanofabrication and puts constraints on possible outcomes. In this work we explore a novel degree of freedom for manipulating the phase by introducing an asymmetric material composition [24] , [25] , [26] . As a proof of principle, we experimentally realize a planar nano-optical antenna in the form of a bimetallic particle dimer and show that it exhibits prominent colour routing properties; that is, it is able to sort light of different colours into different scattering directions. The additive phase accumulation provided through the bimetallic composition makes it possible to achieve this result for an antenna that is deep subwavelength in size, something that is difficult or impossible in previously reported colour routing schemes, including those based on plasmonic particle on a film systems [27] , [28] metal grating structures [29] , [30] , [31] or plasmonic holography [32] . Moreover, we show that dense assemblies of bimetallic colour routers can be fabricated over large areas using cheap colloidal lithography. This may facilitate applications in, for example, optical sensor development, spectroscopy and photonics. 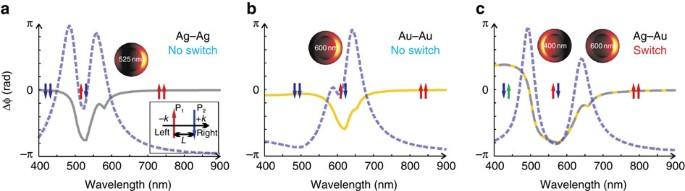Figure 1: Comparison of the relative phase shift between the two resonances in a bimetallic Ag–Au dimer and its monometallic counterparts. Full lines show relative phase shift, while dashed lines show scattering cross-sections versus wavelength. Inset in (a) shows the model system, consisting of a pair of dipoles oriented parallel to each other and separated by a distanceL=120 nm. The particles were modelled using the coupled dipole approximation34and size-corrected dipole polarizabilities for oblate spheroids (a=b=50(65) nm andc=10 nm) using tabulated metal permittivities41. In the monometallic cases, shown in panels (a,b), the phase drops only at wavelengths in between the plasmon resonances of the dipoles, whereas in the bimetallic dimer, (c), the phase first drops and then changes sign due to a mismatch in the permittivity between the two particles. Red and blue arrows indicate the orientation of the dipole moments induced on the particles. The green arrow indicates inversion of the dipole due to interband transitions. Circular insets in (a–c) show radiation patterns (angular resolved scattering diagrams) calculated at the antisymmetric mode frequencies (labelled inside each of the circles) and assuming particle pairs supported on an air–glass interface. The contrast varies from zero intensity dark regions to maximum intensity bright regions. Radial coordinate of the radiation pattern scales as numerical aperture NA=nsinθ and tangential as angleϕ, with angles θ andϕhaving standard spherical coordinate meaning. Two point dipole system To illustrate the idea, we show in Figure 1 an analytical simulation of two weakly interacting induced electric dipoles in metal particles (inset of Fig. 1a ). We consider metal spheroids of slightly different aspect ratio, and therefore different plasmon resonance wavelengths [33] , [34] . The centre-to-centre separation is set to L =120 nm. To see how to achieve directional scattering from an asymmetric dimer, we focus on light scattered in opposite directions along a line connecting the two oscillating particle dipoles. The optical intensity along this line is given by a sum of the individual dipole contributions and an interference term. The latter is proportional to cos( kL +Δ ϕ ), where k is the free space wave vector and Δ ϕ denote an internal phase shift between the two dipoles. The phase shift is determined by the complex particle polarizabilities and therefore varies with the size, shape and material composition of the particles in accordance with their plasmon resonance characteristics. Directional scattering is obtained if interference is maximized in one direction and/or suppressed in the opposite direction. In the ideal case, we would want the argument of the cosine function to reach the limit of constructive interference ( kL +Δ ϕ =2πm, m =0, ±1, ±2...) for light propagating, for example, to the right along the line through the two particles, whereas perfect destructive interference (− kL +Δ ϕ =π+2πm, m =0, ±1, ±2...) is achieved for light propagating to the left. Clearly, this requires that the internal phase shift, Δ ϕ , is different from zero. As shown in Figure 1 , this is indeed possible because of the different sizes and/or material composition of the spheroids, which makes their plasmon resonances occur at separate wavelengths. There is, however, an important difference between the monometallic and bimetallic dimers: in the monometallic cases, a negative phase shift is generated at wavelengths in between the plasmon resonances, but in the bimetallic case, there is an additional positive phase shift in the blue region of the spectrum. Thus, a bimetallic dimer should be able to scatter light of different wavelengths in different directions! This is the basic idea behind our directional colour router. At a fundamental level, the additional phase shift is caused by differences in permittivity between gold (Au) and silver (Ag), in particular, the fact that Au, but not Ag, supports the so-called interband transitions for photon wavelengths between ∼ 400 nm and ∼ 500 nm, which lead to an increase of the imaginary part of the permittivity. Figure 1: Comparison of the relative phase shift between the two resonances in a bimetallic Ag–Au dimer and its monometallic counterparts. Full lines show relative phase shift, while dashed lines show scattering cross-sections versus wavelength. Inset in ( a ) shows the model system, consisting of a pair of dipoles oriented parallel to each other and separated by a distance L =120 nm. The particles were modelled using the coupled dipole approximation [34] and size-corrected dipole polarizabilities for oblate spheroids ( a = b =50(65) nm and c =10 nm) using tabulated metal permittivities [41] . In the monometallic cases, shown in panels ( a,b ), the phase drops only at wavelengths in between the plasmon resonances of the dipoles, whereas in the bimetallic dimer, ( c ), the phase first drops and then changes sign due to a mismatch in the permittivity between the two particles. Red and blue arrows indicate the orientation of the dipole moments induced on the particles. The green arrow indicates inversion of the dipole due to interband transitions. Circular insets in ( a–c ) show radiation patterns (angular resolved scattering diagrams) calculated at the antisymmetric mode frequencies (labelled inside each of the circles) and assuming particle pairs supported on an air–glass interface. The contrast varies from zero intensity dark regions to maximum intensity bright regions. Radial coordinate of the radiation pattern scales as numerical aperture NA= n sinθ and tangential as angle ϕ , with angles θ and ϕ having standard spherical coordinate meaning. 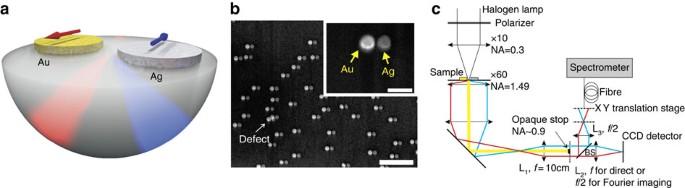Figure 2: Design fabrication and experimental demonstration of bimetallic colour router. (a) An artist's view of colour routing from a bimetallic dimer supported by a glass substrate. (b) Low- and high (inset)-magnification scanning electron microscopy images of bimetallic dimers produced by hole–mask colloidal lithography. Scale bar is 1 μm (inset: 200 nm). (c) Scheme of the experimental setup. White light from a halogen lamp passes through a polarizer and is loosely focused on the sample at normal incidence. The directly transmitted light is effectively filtered out by an opaque stop in the Fourier plane, while light scattered by the dimers at angles higher than the stop (NA∼0.9) passes through to the detectors, a fibre-coupled spectrometer and a charge-coupled device camera. Full size image Realization of a bimetallic nanophotonic colour router As illustrated by the cartoon in Figure 2a , we experimentally demonstrated colour routing using bimetallic dimers composed of pairs of closely spaced silver and gold disks on glass substrates. The dimers were made through evaporation of Au and Ag through a mask with circular holes using a variant of hole–mask colloidal lithography [35] . The two metals are deposited sequentially using two different evaporation angles on opposite sides of the substrate normal so that two closely spaced metal disks are produced. Figure 2b shows scanning electron microscopy images of the resulting bimetallic dimers. The method allows for fabrication of dimers over substantial areas (wafer scale) while preserving the structure orientation, size and composition. The inset shows a magnified view of a dimer. The different contrast of the right and left disks assures that these are indeed Ag and Au particles, in accordance with the design. The diameters of the Au disks were about 130 nm, whereas the Ag disks were slightly smaller, about 110 nm in diameter, because they were evaporated at a later stage. The gap between the particles was ∼ 15 nm. The overall volume of a single dimer, thus, does not exceed a value of approximately ∼ λ 3 /100, where λ is the wavelength of visible light. In addition, some dimers overlapped due to aggregated polystyrene beads used to produce the mask. These defect sites ( Fig. 2b ) slightly reduce the directionality of the scattered light, but fortunately they occur only rather rarely. Figure 2: Design fabrication and experimental demonstration of bimetallic colour router. ( a ) An artist's view of colour routing from a bimetallic dimer supported by a glass substrate. ( b ) Low- and high (inset)-magnification scanning electron microscopy images of bimetallic dimers produced by hole–mask colloidal lithography. Scale bar is 1 μm (inset: 200 nm). ( c ) Scheme of the experimental setup. White light from a halogen lamp passes through a polarizer and is loosely focused on the sample at normal incidence. The directly transmitted light is effectively filtered out by an opaque stop in the Fourier plane, while light scattered by the dimers at angles higher than the stop (NA ∼ 0.9) passes through to the detectors, a fibre-coupled spectrometer and a charge-coupled device camera. Full size image Figure 2c gives a schematic of the experimental setup. Our detection scheme relies on effective discrimination between the scattered and directly transmitted fields by an opaque stop installed in a secondary back-focal plane of the microscope system. Note that this does not significantly affect the light scattered from the dimers positioned on top of the air–glass interface, because most of the scattering is emitted at angles exceeding the critical angle of the interface, that is, at NA>1 (sometimes this light is referred as the forbidden light) [36] , [37] , [38] . The directly transmitted incident radiation, on the other hand, is completely blocked by the opaque stop. The experimental setup is able to record both direct and back-focal plane Fourier images, as well as spectroscopic data for a selected solid angle. The sample was excited with loosely focused, linearly polarized, white light from the air side. A sample area with a diameter of the order 100 μm is excited, which means that thousands of dimers contribute to the overall signal. However, as individual dimers are far apart and the sample lacks long-range spatial order due to the fabrication process, the measured signal can be thought of as a simple sum of individual dimer contributions. 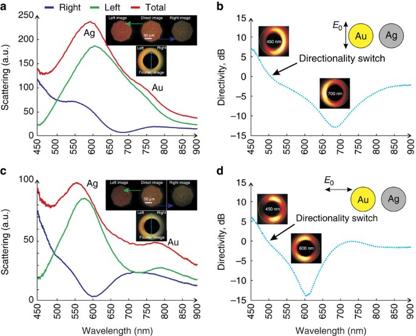Figure 3: Experimental scattering and directivity measurements. Results obtained for incident polarization perpendicular (a,b) and parallel (c,d) to the dimer axis. Panels (a) and (c) summarize spectra collected in right (blue) and left (green) directions, as well as the sum in those two channels (red). Insets show corresponding direct and Fourier colour images. Directional emission is clearly observed for both polarization configurations. Panels (b) and (d) further confirm this through radiation patterns recorded at specific wavelengths corresponding to scattering to the right (450 nm) and to the left (700 nm or 600 nm) as well as through experimental directivities as a function of wavelength. Figure 3 summarizes the experimental results. The insets in Figure 3a show colour images of the sample excited with white light polarized perpendicular to the dimer axis. This excitation corresponds to the scheme proposed in Figure 1 . Right and left directions were arbitrary chosen to correspond to emission towards the Ag and Au particles, respectively. One clearly sees that the colour in the right part of the Fourier image is blue-green, while it is more reddish in the left part. The left and right channels are separated by an imaginary vertical line (blue dotted in the Figure 3a,c through the centre of the Fourier plane). Right and left direct images were obtained by covering the complementary Fourier channel with an opaque screen. It is evident even to the naked eye that the colours of the images are different. The corresponding spectra show this in more detail. Two broad plasmon resonances of Ag ( ∼ 600 nm) and Au ( ∼ 750 nm) are easily identified and one finds a switching point between preferential scattering to the right and to the left at around 500 nm. Plotting the wavelength dependent directionality measured in decibels gives a more quantitative illustration of the colour routing effect. As shown in Figure 3b , the directivity reverts at around 500 nm and reaches maxima of +7 at around 450 nm and −12 at around 680 nm. Fourier images (see inset in Fig. 3b ) recorded at 450 nm and 700 nm using 40 nm bandwidth transmission filters further confirm switching of the directionality. Those images together with the very high directivities constitute direct experimental evidence for highly wavelength dependent directional scattering, or colour routing, from bimetallic dimers. Figure 3: Experimental scattering and directivity measurements. Results obtained for incident polarization perpendicular ( a,b ) and parallel ( c,d ) to the dimer axis. Panels ( a ) and ( c ) summarize spectra collected in right (blue) and left (green) directions, as well as the sum in those two channels (red). Insets show corresponding direct and Fourier colour images. Directional emission is clearly observed for both polarization configurations. Panels ( b ) and ( d ) further confirm this through radiation patterns recorded at specific wavelengths corresponding to scattering to the right (450 nm) and to the left (700 nm or 600 nm) as well as through experimental directivities as a function of wavelength. Full size image Figure 3c,d shows the same kind of experiment as in Figure 3a,b , but performed with the incident polarization parallel to the dimer axis. In this case, the Fourier image also looks asymmetric in the right and left directions and the direct images show clear colour differences. Fourier images recorded at 450 nm and 600 nm (inset in Fig. 3d ) again confirm the colour routing effect. Note that the Ag peak is blue-shifted ( ∼ 560 nm), while the Au peak is red-shifted ( ∼ 800 nm) compared with the perpendicular polarization case. These shifts are due to the increased near-field dipole-dipole coupling between the particles in each dimer [26] and clearly affects the positions of directivity extrema, with the left maximum now occurring at around 620 nm (directivity ≈ −12 dB). The data thus suggest that the incident polarization provides a powerful way to tune the spectral response of the colour routing effect. To provide additional evidence that the colour routing effect is indeed an intrinsic property of each individual bimetallic dimer, we performed full electrodynamic simulations using the Green's function method for stratified media [39] , [40] . Two disks, both with diameter 100 nm and thickness 40 nm, were positioned on an air–glass interface with a gap distance of 20 nm. 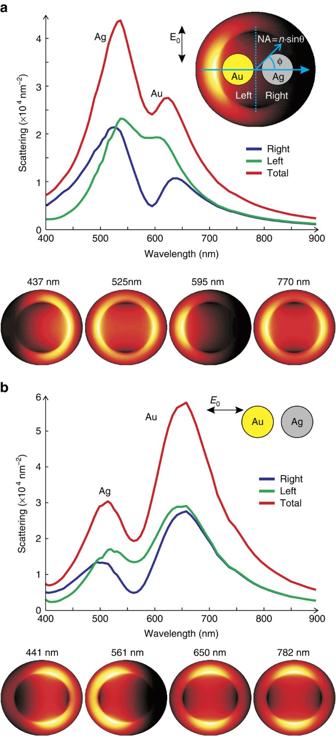Figure 4: Full electrodynamic simulation of wavelength specific directional light scattering from a bimetallic dimer. (a) Gold and silver disks (100 nm wide and 40 nm high) separated by a 20-nm gap and excited at normal incidence with light polarization perpendicular to the dimer axis. (b) The same dimer with light polarization parallel to the dimer axis. (a) The spectra correspond to light scattered within the glass hemisphere to the right (blue), left (green) and the sum the two (red). Right and left spectra are integrated over −π/2<ϕ<π/2 and π/2<ϕ<3π/2, respectively. Inset shows orientation of dimer with respect to the radiation pattern. Radial coordinate of the radiation pattern scales as numerical aperture NA=nsinθ and tangential as angleϕ. Simulated Fourier images at specific wavelengths. The radiation pattern in (a) shows clear transitions from directional colour routing at 437 nm and 595 nm to nearly symmetric scattering at 525 and 770 nm. In (b), similar behaviour is observed at 441 nm and 561 nm, with the directivity maximum slightly shifted to blue. The orientation of the disks and the polarization configuration is the same as in Figure 3 , that is, the incident field enters from the air side and is polarized perpendicular to the dimer axis in Figure 4a and parallel to it in Figure 4b . The scattered light was then integrated over directions within the glass half-space, with right and left directions corresponding to emission towards the Ag and Au particles, respectively. The spectra in Figure 4a,b show that the simulations are in excellent overall agreement with the experimental data. Referring back to the simple dipole picture in Figure 1 , there are two distinct peaks, associated with the Au- and Ag-localized dipolar plasmon resonances. At wavelengths longer than ∼ 700 nm, to the red of both resonances, the intensities in both channels are the same, but for wavelengths between two resonances, where the two dipoles are out of phase, the left channel dominates. This is especially evident in the radiation pattern at 595 nm plotted at the bottom of Figure 4a . Finally, at wavelengths shorter than 500 nm, to the blue of both resonances, we clearly see a reverse in the emission direction. This is due to the interband transitions in Au and the fact that the Ag dipole moment now lags the driving field. The lower panels of Figure 4a,b show radiation patterns for four different wavelengths, again confirming that a single bimetallic dimer can scatter light preferably in either the right or left direction depending on the wavelength of excitation. Corresponding magnitudes and phases of total dipole moments induced in Au and Ag disks are shown in Supplementary Figure S1 . Figure 4: Full electrodynamic simulation of wavelength specific directional light scattering from a bimetallic dimer. ( a ) Gold and silver disks (100 nm wide and 40 nm high) separated by a 20-nm gap and excited at normal incidence with light polarization perpendicular to the dimer axis. ( b ) The same dimer with light polarization parallel to the dimer axis. ( a ) The spectra correspond to light scattered within the glass hemisphere to the right (blue), left (green) and the sum the two (red). Right and left spectra are integrated over −π/2< ϕ <π/2 and π/2< ϕ <3π/2, respectively. Inset shows orientation of dimer with respect to the radiation pattern. Radial coordinate of the radiation pattern scales as numerical aperture NA= n sinθ and tangential as angle ϕ . Simulated Fourier images at specific wavelengths. The radiation pattern in ( a ) shows clear transitions from directional colour routing at 437 nm and 595 nm to nearly symmetric scattering at 525 and 770 nm. In ( b ), similar behaviour is observed at 441 nm and 561 nm, with the directivity maximum slightly shifted to blue. Full size image In summary, we have demonstrated that a bimetallic particle dimer as small as ∼ λ 3 /100 can function as a nanophotonic colour router. The effect originates in optical phase shifts induced through the asymmetric material composition of the dimer. We have here focused on dimers composed of Au and Ag particles, but the concept is not limited to these materials. Other pairs of metals with appropriate wavelength-dependent permittivities, for example, aluminium—copper dimers, should also be suitable for colour routing. The concept is also restricted neither to disk-shaped particles nor to a horizontal arrangement of the dimers. Indeed, by optimizing the shape, size and orientation of the individual particles in a bimetallic dimer, it is likely that much higher wavelength and polarization-dependent directivities than observed here can be achieved. On the other hand, the simple material-induced symmetry breaking used here does not require careful size optimization or use of special geometries, thereby facilitating nanofabrication. We believe that our findings can significantly broaden the versatility of plasmonic devices and we envision possible practical implementations in meta-materials, directional emitters, photon couplers and sorters and in chemo-/bio-sensors. Point dipole simulations Each particle in the dimer systems shown in Figure 1 was assumed to be a metal spheroid made of Au or Ag with dipole polarizabilities given by: [33] Here i = x , y , z , a , b and c are the spheroid semiaxes, ɛ m(d) are the complex permittivities of the metals, modelled using data from Johnson and Christy [41] , and the surrounding dielectric medium, respectively, and f i are geometrical shape factors satisfying f x + f y + f z =1. The polarizabilities were corrected for finite-size effects by using the so-called modified long wavelength approximation and interparticle coupling was modelled through the coupled dipole approximation [34] . The particles were assumed to be oblate spheroids of slightly different sizes with semiaxes a = b =50(65) nm and c =10 nm. Green's function method For calculation of scattering spectra and radiation patterns in Figure 4 we used the Green's function method [39] , [40] , with cubic mesh elements of 2 nm side. Right and left spectra were calculated by integrating over a corresponding half of the Fourier plane in glass. Fabrication of bimetallic dimers Au–Ag heterodimer nanoantennas were fabricated using so-called hole–mask colloidal lithography [35] . After preparing the colloidal mask, which defines the size of the nanodisks, Au and Ag were evaporated sequentially at an angle of 25° and −25°, respectively. By varying the evaporation angle, one can control the separation between particles in the dimer, whereas the evaporation time and rate defines the thickness of the disks. Electron microscopy Scanning electron microscopy images were taken with a JEOL JSM-6301F microscope at an acceleration voltage of 10 keV. Low-vacuum mode imaging significantly reduced charging problems associated with the non-conductive glass substrates. The contrast in the secondary electron detector is proportional to the atomic number, which means that the bright disks seen in Figure 2 correspond to Au and the darker to Ag nanoparticles, in accordance with the design. Optical spectroscopy Optical excitation of the Au–Ag dimers was performed using linearly polarized white light from a halogen lamp (100 W) focused by a low NA lens from the air side. The sample was mounted on the XY stage of an inverted microscope (Nikon TE-2000E) equipped with an ultrahigh NA oil immersion objective (X60 NA=1.49, Nikon). Fourier images were obtained by means of an achromatic 4 f correlator scheme, whereas the spectra were recorded by a fibre-coupled grating spectrometer [38] . The incident radiation was blocked from reaching the detector by an opaque stop installed in the secondary Fourier plane. The opaque stop had a diameter that corresponded to NA<0.9, so that the light emitted at higher angles could pass through. To record right and left images, the corresponding half of the secondary Fourier plane was covered with an additional opaque screen. Directional spectra were recorded by positioning the collection fibre of the spectrometer in the Fourier plane. The 'right' channel was collected at an angle corresponding to NA ∼ 1.2 in the direction of silver ( ϕ =0) while the 'left' channel was collected at the same angle but in the direction of Au ( ϕ =180). How to cite this article: Shegai, T. et al . A bimetallic nanoantenna for directional colour routing. Nat. Commun. 2:481 doi: 10.1038/ncomms1490 (2011).